Visualizing the replication of respiratory syncytial virus in cells and in living mice Respiratory syncytial virus (RSV) is the most important cause of severe lower-respiratory tract disease in calves and young children, yet no human vaccine nor efficient curative treatments are available. Here we describe a recombinant human RSV reverse genetics system in which the red fluorescent protein (mCherry) or the firefly luciferase (Luc) genes are inserted into the RSV genome. Expression of mCherry and Luc are correlated with infection rate, allowing the monitoring of RSV multiplication in cell culture. Replication of the Luc-encoding virus in living mice can be visualized by bioluminescent imaging, bioluminescence being detected in the snout and lungs of infected mice after nasal inoculation. We propose that these recombinant viruses are convenient and valuable tools for screening of compounds active against RSV, and can be used as an extremely sensitive readout for studying effects of antiviral therapeutics in living mice. Human respiratory syncytial virus (HRSV) is the main cause of bronchiolitis and pneumonia among infants and children under 1 year of age worldwide, and the major cause of hospitalization during infancy [1] . There is currently no vaccine available against HRSV, and antiviral treatments are limited to the use of Synagis (palivizumab), an expensive humanized monoclonal antibody only used as a preventive treatment, and ribavirin, a nucleoside antimetabolite having severe toxicological liabilities and that is used under exceptional circumstances. There is therefore an urgent need for discovering new molecules capable of inhibiting RSV replication. Together with bovine RSV, canine pneumovirus [2] and pneumovirus of mice, HRSV belongs to the genus Pneumovirus of the family Paramyxoviridae , order Mononegavirales [3] . RSV is an enveloped nonsegmented negative-stranded RNA virus with a 15-kb genome that is transcribed into 10 subgenomic messenger RNAs (mRNAs) that encode 11 proteins, including the 4 proteins of the nucleocapsid, N, P, L and M2-1, and the attachment G and fusion F surface glycoproteins that are the major neutralization and protective antigens. The gene order is 3′- NS1-NS2-N-P-M-SH-G-F-M2-L -5′. The genome of RSV possesses a single polymerase entry site for transcription at the 3′ end in the leader region, and transcription of the genes occurs in a sequential polar fashion from 3′ to 5′. There is thus a gradient of transcription from 3′ to 5′ and the level of each RSV mRNA correlates with its distance from the 3′ promoter in the genome, that is, the 3′-most gene gives rise to the greatest amount of mRNA [4] , [5] . The nonstructural NS1 and NS2 genes are the first to be transcribed and are the most abundant. These genes encode proteins that target the cellular antiviral response, thus their rapid and strong expression is crucial for virus survival, as soon as the RSV nucleocapsid has penetrated into the cytoplasm. The search for RSV inhibitors is generally based on laborious, time-consuming and expensive methods, which generally consist in the analysis of cytopathic effect by microscopy, reduction of virus replication by immunostaining, plaque reduction assays, quantitative reverse transcriptase (qRT)-PCR, enzyme-linked immunosorbent assay tests or reduction of RSV-induced cell cytotoxicity. Viruses with modified genomes and expressing reporter genes, such as those coding for the green fluorescent protein (GFP) or luciferase, are more suitable for such screenings. Coupled to the use of automated plate readers, reporter gene-carrying recombinant viruses can make these assays more suitable for standardization and high-throughput purposes. Infectious recombinant HRSV (rHRSV) can be produced by intracellular co-expression from transfected plasmids of an RSV antigenomic RNA, which is the positive-sense replicative intermediate of genomic RNA, together with the N, P, M2-1 and L proteins [6] . Modelling HRSV disease in vivo is an indispensable step in the search for novel therapies and preventive measures for HRSV disease. So far, methods for monitoring the course of infection with RSV in real time in living animals are lacking. The most common experimental non-primate models of HRSV infection are rodent models, including inbred BALB/c mice and cotton rats [7] . Following HRSV infection, viral load usually peaks by the fourth day and wanes by the eighth day. Viral load is generally estimated by qRT-PCR using RNA extracted from homogenized lung tissue of infected animals, which is laborious and time consuming. Genetically engineered RSV expressing either GFP , beta-galactosidase , Katushka or Renilla luciferase foreign genes were previously constructed [8] , [9] , [10] , [11] , however, there is no report for their use in vivo . Several recombinant viruses expressing luciferase genes, such as Sendai virus [12] , Sindbis virus [13] , dengue virus [14] , vaccinia virus [15] , herpes simplex virus [16] , human adenovirus [17] , mouse coronavirus [18] and influenza virus [19] have been engineered for in vivo studies previously. Here we describe the engineering of new rHRSVs, derived from the strain Long, expressing either the firefly luciferase (Luc) or the mCherry red fluorescent proteins and their use as tools for antiviral screening when combined to automated fluorescent plaque counting. To avoid any negative effect on the expression of the NS genes, the reporter genes were placed between P and M genes. Furthermore, we report the visualization of HRSV infection in living mice using the rHRSV carrying the Luc reporter gene, a new approach for real-time study of RSV infection and evaluation of antiviral therapeutics in vivo . Construction and rescue of rHRSV vectors Our first goal was to engineer a complementary DNA (cDNA) copy of the HRSV genome carrying unique restriction enzyme sites located in intergenic regions to facilitate further manipulations of the RSV genome and modification of individual genes. In addition to the XhoI and BamHI sites that were naturally present in the end of the SH gene and the beginning of the L gene, respectively, seven unique sites were introduced in intergenic regions, and one (SalI) in the variable region 2 of L [21] . Eleven segments covering the entire RSV genome were individually amplified, cloned and sequentially assembled in a low-copy pACNR1180 vector [22] ( Fig. 1a ). A T7 RNA polymerase promoter was placed upstream the Leader region such that antigenomic RNA would be transcribed with three supplementary G residues at the 5′ end. The hepatitis delta virus (HDV) antigenome ribozyme sequence was fused to the last nucleotide of the trailer sequence to achieve correct cleavage. 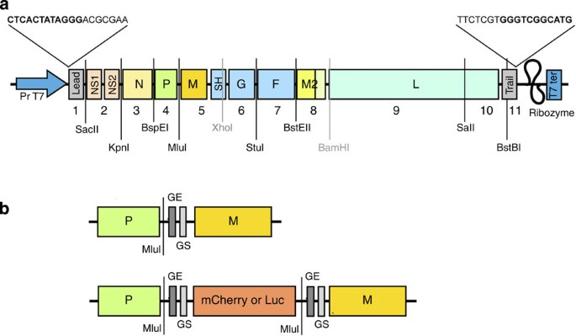Figure 1: Schematic of construction of infectious clones derived from HRSV Long strain. (a) Genome map of antigenomic cDNA construction (not to scale). Protein-encoding frames are shown as coloured boxes, leader and trailer regions as grey boxes. Intergenic regions are shown as a black horizontal line. The HDV ribozyme is shown as a curved black line and the T7 transcription terminator as a small blue box. The sequences of junctions between the T7 promoter (arrow) and the leader sequence, and between the HDV ribozyme (curved line) and the trailer sequence are shown in the enlargements. The 11 DNA fragments that were assembled are numbered as inTable 1. The full-length HRSV cDNA was assembled into a reverse genetic vector using additional restriction sites introduced in the intergenic regions (in black) or naturally present in the HRSV genome sequence (in grey). The SalI cleavage site introduced in theLgene was silent at the amino-acid level. (b) ThemCherryorfirefly luciferasegene was inserted betweenPandMgene together with an upstream gene end (GE) and a downstream gene start (GS) signals as described in Methods. Figure 1: Schematic of construction of infectious clones derived from HRSV Long strain. ( a ) Genome map of antigenomic cDNA construction (not to scale). Protein-encoding frames are shown as coloured boxes, leader and trailer regions as grey boxes. Intergenic regions are shown as a black horizontal line. The HDV ribozyme is shown as a curved black line and the T7 transcription terminator as a small blue box. The sequences of junctions between the T7 promoter (arrow) and the leader sequence, and between the HDV ribozyme (curved line) and the trailer sequence are shown in the enlargements. The 11 DNA fragments that were assembled are numbered as in Table 1 . The full-length HRSV cDNA was assembled into a reverse genetic vector using additional restriction sites introduced in the intergenic regions (in black) or naturally present in the HRSV genome sequence (in grey). The SalI cleavage site introduced in the L gene was silent at the amino-acid level. ( b ) The mCherry or firefly luciferase gene was inserted between P and M gene together with an upstream gene end (GE) and a downstream gene start (GS) signals as described in Methods. Full size image To develop a simple, fast and high-throughput antiviral assay against RSV, we then inserted the gene coding for the monomeric red fluorescent protein mCherry or firefly luciferase ( Luc ), flanked by RSV gene start and gene end signals into the Mlu I site located between P and M genes ( Fig. 1b ). The recombinant rHRSV-Cherry and rHRSV-Luc thus expressed one additional mRNA, namely mCherry or Luc, compared with rHRSV. These plasmids were transfected into BSRT7/5 cells along with four other plasmids encoding the N, P, L and M2-1 proteins to support RSV transcription and replication, as previously described [6] . Viable recombinant viruses were recovered from all three cDNA constructs. The multicycle growth competence of the recombinant viruses from passage 3 was compared with wild-type (WT) HRSV. As shown in Fig. 2a , growth kinetics of recombinant viruses were not significantly different compared with WT parental HRSV (three independent experiments, two-way analysis of variance on logarithmic-transformed data). For all viruses, maximum titres were observed at 48 h post infection (p.i.) with titres of 6.33±0.25 Log plaque forming units (p.f.u.) ml −1 for HSRV Long strain, 6.12±0.48 Log p.f.u. ml −1 for rHRSV, 5.92±0.53 Log p.f.u. ml −1 for rHRSV-mCherry and 5.82±0.25 Log p.f.u. ml −1 for rHRSV-Luc. The plaque phenotypes of parental and recombinant viruses shown in Fig. 2c appeared also very similar: plaque diameters were measured and no significant differences were observed ( Supplementary Table 1 ). The mCherry fluorescence was readily detectable at 24 h p.i. in HEp-2 cells using a fluorescent plate reader ( Fig. 2d ) or a fluorescence microscope ( Fig. 2b ), and fluorescence steadily increased at 48 h and 72 h ( Fig. 2d ). Luciferase activity was also detectable in extracts from infected cells from 24 to 72 h p.i. ( Fig. 2d ). The signal-to-noise ratio was higher for luciferase compared with mCherry (see below). Viruses present in the cell supernatants were then propagated by three passages on HEp-2 cells. Expression of the mCherry or Luc reporter was shown to be stable over the course of eight passages. Thus, insertion of mCherry or Luc reporter genes between P and M genes has no major impact on the replicative capacities of the virus. 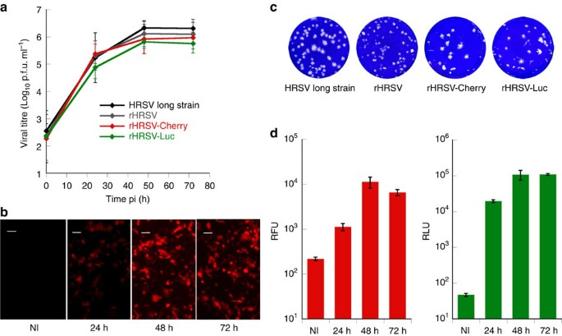Figure 2: Growth properties of recombinant HRSV viruses. (a) Growth curves of the parental HRSV Long strain, the wild-type recombinant HRSV (rHRSV) and the recombinant HRSV expressing mCherry (rHRSV-Cherry) or firefly luciferase (rHRSV-Luc) on HEp-2 cells. Cell monolayers were infected at an MOI of 0.01 and incubated at 37 °C. At the indicated time points, viruses were harvested and titrated by plaque assays on HEp-2 cells. (b) Fluorescent images of HEp-2 cells infected with rHRSV-Cherry at an multiplicity of infection (MOI) of 0.01 at the indicated time points after infection observed in an inverted fluorescence microscope. Original magnification × 200; bar, 50 μm. (c) Plaque phenotypes of the HRSV Long strain and the recombinant rHRSV, rHRSV-Cherry and rHRSV-Luc assayed on HEp-2 cells, as described in Methods. Cell monolayers were stained with crystal violet after 6 days of incubation at 37 °C. Representative data are shown. The viral stocks used for infection were diluted 104-fold for this plaque assay. (d) For rHRSV-Cherry and rHRSV-Luc, red fluorescence (red bars) and luminescence (green bars) were measured respectively at indicated time points after infection at an MOI of 0.01. The results are expressed as mean±s.d. for three independent experiments performed in triplicate. NI, non-infected; RFU, relative fluorescence units; RLU, relative light units. Figure 2: Growth properties of recombinant HRSV viruses. ( a ) Growth curves of the parental HRSV Long strain, the wild-type recombinant HRSV (rHRSV) and the recombinant HRSV expressing mCherry (rHRSV-Cherry) or firefly luciferase (rHRSV-Luc) on HEp-2 cells. Cell monolayers were infected at an MOI of 0.01 and incubated at 37 °C. At the indicated time points, viruses were harvested and titrated by plaque assays on HEp-2 cells. ( b ) Fluorescent images of HEp-2 cells infected with rHRSV-Cherry at an multiplicity of infection (MOI) of 0.01 at the indicated time points after infection observed in an inverted fluorescence microscope. Original magnification × 200; bar, 50 μm. ( c ) Plaque phenotypes of the HRSV Long strain and the recombinant rHRSV, rHRSV-Cherry and rHRSV-Luc assayed on HEp-2 cells, as described in Methods. Cell monolayers were stained with crystal violet after 6 days of incubation at 37 °C. Representative data are shown. The viral stocks used for infection were diluted 10 4 -fold for this plaque assay. ( d ) For rHRSV-Cherry and rHRSV-Luc, red fluorescence (red bars) and luminescence (green bars) were measured respectively at indicated time points after infection at an MOI of 0.01. The results are expressed as mean±s.d. for three independent experiments performed in triplicate. NI, non-infected; RFU, relative fluorescence units; RLU, relative light units. Full size image To establish settings on the equipment required for automated plaque counting, we used several dilutions of rHRSV-Cherry and rHRSV-Luc to infect HEp-2 cells in 96-well plates, and automated counting of fluorescence and luminescence was done at different times. Representative data are shown in Fig. 3 . Dose–response curves expressed in terms of the response (relative light units (RLUs) or relative fluorescence units on a logarithmic scale) versus the dose (p.f.u. per well on a logarithmic scale) demonstrated a broad linear dynamic range between 1,000 and 50 p.f.u. per well for rHRSV-Cherry, and between 3,000 and 5 p.f.u. for rHRSV-Luc. The best dynamic range was observed 24 h p.i. for rHRSV-Luc, while the rHRSV-mCherry fluorescent signal was higher at 48 h p.i.. For both viruses the signals were more variable and even decreased after 72 h of infection, probably due to viral cytopathic effect. The dynamic was better for Luc compared with mCherry, with linear RLU values extending over >3 orders of magnitude (log 10 ). There was a strong correlation between the viral dose and luciferase activity. From these results, inocula of 500 and 1,000 p.f.u. per well of 96-well plates were then used for further assays for rHRSV-Cherry and rHRSV-Luc, respectively, and fluorescence and luminescence were read at 48 h p.i. and 24 h p.i., respectively (arrows in Fig. 3a,b ). 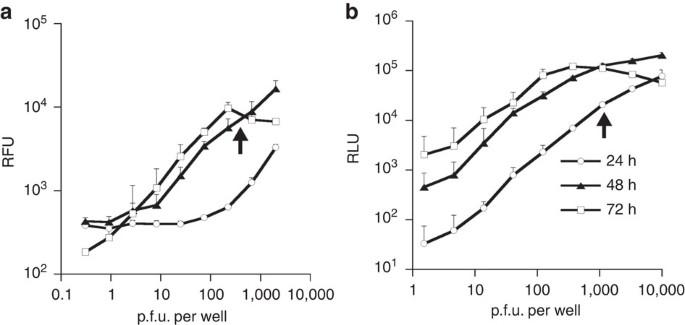Figure 3: Correlation between input virus titres, fluorescence and luminescence at different times post infection. Scatter plots of automatic counting of fluorescence of rHRSV-Cherry (a) and rHRSV-Luc luminescence (b) (Yaxis) measured at different times post infection, as indicated with defined amounts of input virus. The results are expressed as mean value+s.d. of two independent experiments performed in triplicate. Black arrows indicate the signal at the time end point and the viral input chosen for further experiments. Figure 3: Correlation between input virus titres, fluorescence and luminescence at different times post infection. Scatter plots of automatic counting of fluorescence of rHRSV-Cherry ( a ) and rHRSV-Luc luminescence ( b ) ( Y axis) measured at different times post infection, as indicated with defined amounts of input virus. The results are expressed as mean value+s.d. of two independent experiments performed in triplicate. Black arrows indicate the signal at the time end point and the viral input chosen for further experiments. Full size image Using rHRSV-Cherry and rHRSV-Luc for antiviral screenings To validate that rHRSV-Cherry and rHRSV-Luc can be used as tools for high-throughput antiviral screens, HEp-2 cells were infected either with rHRSV-Cherry or with rHRSV-Luc in the presence of the RSV L polymerase inhibitor AZ-27 or the RSV fusion inhibitor BMS-433771 analogue (AZD4316) [23] . Serially diluted inhibitors were added to viral inocula and incubated on HEp-2 cells for 24 (luminescence) or 48 h (fluorescence). Luciferase and mCherry signals were measured to assess inhibition of viral replication. Both fluorescence and luminescence signals decreased while increasing RSV inhibitor concentrations, whereas control dimethyl sulfoxide (DMSO) had no effect ( Fig. 4a,b ). Effect of compounds on mCherry expression in rHRSV-Cherry-infected cells is obvious using a fluorescence microscope ( Fig. 4c ) and is measurable with a fluorescent plate reader ( Fig. 4b ). Reduction of luciferase activity ( Fig. 4a ) or mCherry fluorescence ( Fig. 4b ) in rHRSV-Luc- or rHRSV-Cherry-infected cells treated with the two compounds allowed the determination of the half maximal effective concentration (EC 50 ) values for both inhibitors. For AZD4316, the observed EC 50 values were 1.0 nM for rHRSV-Cherry and 1.7 nM for rHRSV-Luc, consistent with its EC 50 of 2–40 nM against different HRSV strains in a 3-day infection assay [23] . For AZ-27, the observed EC 50 values were 28 and 38 nM with rHRSV-Cherry and rHRSV-Luc, respectively, similar to the published EC 50 of about 10 nM with HRSV strain A2 (refs 25 , 26 ). To compare this method with a classical method, the EC 50 of AZ-27 and AZD4316 were also determined by the plaque reduction assay using rHRSV ( Fig. 4d ). The observed EC 50 , 14 and 0.6 nM for AZ-27 and AZD4316, respectively, were in the same range as those determined by luminescent or fluorescent assays. The 50% cytotoxic concentration values obtained with HEp-2 cells, >250 μM for AZ-27 and about 50 μM for AZD4316, were much higher than the EC 50 values. 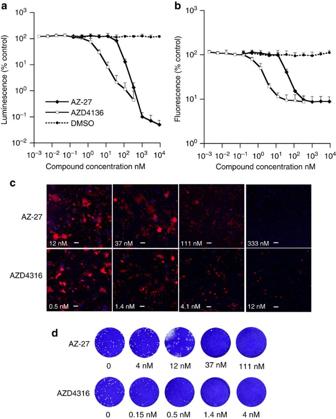Figure 4: Inhibition of rHRSV-mCherry and rHRSV-Luc replication by AZ-27 and AZD4136 compounds. HEp-2 cells in 96-well plates were infected with 1,000 p.f.u. of rHRSV-Luc (a) or 500 p.f.u. of rHRSV-mCherry (b) in the presence of serial dilutions of AZ-27, AZD4316 compounds or control DMSO. (a) The luciferase activity was measured at 24 h post infection using an automatic plate luminometer. (b) The red fluorescence was read at 48 h p.i. by automatic counting and as described in Methods. (c) Visualizing rHRSV-mCherry replication inhibition by fluorescence microscopy. After automatic counting of fluorescence, cells were observed with an inverted fluorescence microscope. Nuclei are stained in blue with Hoechst 33342. Drug concentrations are indicated on the micrograph. Original magnification × 200; bar, 100 μm. (d) The effect of AZ-27 and AZD4316 compounds on rHRSV replication was also analysed by the plaque reduction assay on HEp-2 cells in the presence of the indicated dilutions of AZ-27 and AZD4316 compounds. All shown data are from one experiment representative of three independent experiments performed in triplicate (mean+s.d.). Figure 4: Inhibition of rHRSV-mCherry and rHRSV-Luc replication by AZ-27 and AZD4136 compounds. HEp-2 cells in 96-well plates were infected with 1,000 p.f.u. of rHRSV-Luc ( a ) or 500 p.f.u. of rHRSV-mCherry ( b ) in the presence of serial dilutions of AZ-27, AZD4316 compounds or control DMSO. ( a ) The luciferase activity was measured at 24 h post infection using an automatic plate luminometer. ( b ) The red fluorescence was read at 48 h p.i. by automatic counting and as described in Methods. ( c ) Visualizing rHRSV-mCherry replication inhibition by fluorescence microscopy. After automatic counting of fluorescence, cells were observed with an inverted fluorescence microscope. Nuclei are stained in blue with Hoechst 33342. Drug concentrations are indicated on the micrograph. Original magnification × 200; bar, 100 μm. ( d ) The effect of AZ-27 and AZD4316 compounds on rHRSV replication was also analysed by the plaque reduction assay on HEp-2 cells in the presence of the indicated dilutions of AZ-27 and AZD4316 compounds. All shown data are from one experiment representative of three independent experiments performed in triplicate (mean+s.d.). Full size image Real-time in vivo imaging of RSV infection The recent development of highly sensitive cameras has enabled the use of luciferase reporter viruses for in vivo imaging studies of viral replication and spread. To apply this approach to RSV, we used rHRSV-Luc in an attempt to visualize RSV replication in the mouse model. BALB/c mice were infected with the reporter virus via intranasal (IN) inoculation with 5 × 10 4 p.f.u. and in vivo bioluminescence intensity was determined daily ( Fig. 5a ). Mice were anaesthetized and observed alive using the IVIS imaging system 5 min after IN injection of D -luciferin. Compared with intraperitoneal (IP) injection, IN instillation of luciferin confers a one to two orders of magnitude increase in luciferase bioluminescence detection in both lung and nose [27] ( Supplementary Fig. 1 ). The weight ( Fig. 5b ) and temperature (not shown) of animals were also measured and no signs of morbidity were observed. Bioluminescence was observed in the respiratory tract only, and detected as early as 3 d.p.i. both in the snout and in the lungs of rHRSV-Luc-infected animals. Maximum bioluminescence was observed at 3 d.p.i. in the snout, while light output peaked on days 4 and 5 for lungs and remained detectable for at least 7 days after initiating the infection ( Fig. 5a ). No bioluminescence was observed for mice infected with WT HRSV ( Fig. 5a ). Left and right lungs were equivalently infected ( Supplementary Fig. 2 ). It is remarkable that in our primo-infection experiments with the Long strain, using low amounts of RSV infectious particles, RSV replication was clearly visualized, although no significant weight loss nor other clinical sign was observed with either WT or recombinant rHRSV-Luc virus. To verify that rHRSV-Luc replicated in the respiratory tract only, luciferase activity was quantified on either isolated organs or organ homogenates. As shown in Supplementary Fig. 3 , bioluminescence was observed in isolated lungs, but not in liver or spleen. Luciferase activity was also detected with lung but not in liver and spleen homogenates. 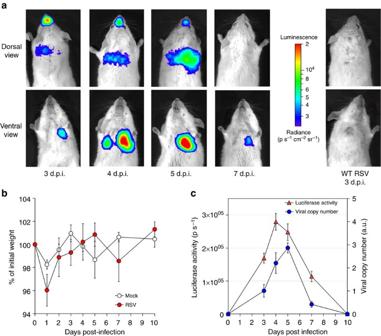Figure 5:In vivoluminescence of rHRSV-Luc-infected mice. (a) Groups of 4 BALB/c mice were infected at day 0 by rHRSV-Luc (5 × 104p.f.u. per mouse). Bioluminescence was then measured daily by intranasal injection of 50 μl ofD-luciferin (200 μM) and capture of photon emission from the chest at different days post infection (d.p.i.) using the IVIS system. Dorsal and ventral views of one mouse representative of the results are shown. The scale on the right indicates the average radiance: the sum of the photons per second from each pixel inside the region of interest/number of pixels (p s−1cm−2sr−1). On the right is shown a mouse infected by WT HRSV and used as a negative control for bioluminescence at 3 d.p.i. (b) Time course of body-weight changes; mice were mock-infected or infected with 6 × 104p.f.u. of rHRSV-Luc and their weights measured every day. (c) Comparison of bioluminescence and viral copy number. Luciferase activities were quantified using ‘Living Image’ software, and quantitative RT-PCR were performed on RNA recovered from mouse lung homogenates. Each data point represents mean±s.e.m. (qRT-PCRn=3; luciferasen=7). Luciferase activity is expressed as p s−1and viral copy number is expressed as arbitrary units (a.u.). Figure 5: In vivo luminescence of rHRSV-Luc-infected mice. ( a ) Groups of 4 BALB/c mice were infected at day 0 by rHRSV-Luc (5 × 10 4 p.f.u. per mouse). Bioluminescence was then measured daily by intranasal injection of 50 μl of D -luciferin (200 μM) and capture of photon emission from the chest at different days post infection (d.p.i.) using the IVIS system. Dorsal and ventral views of one mouse representative of the results are shown. The scale on the right indicates the average radiance: the sum of the photons per second from each pixel inside the region of interest/number of pixels (p s −1 cm −2 sr −1 ). On the right is shown a mouse infected by WT HRSV and used as a negative control for bioluminescence at 3 d.p.i. ( b ) Time course of body-weight changes; mice were mock-infected or infected with 6 × 10 4 p.f.u. of rHRSV-Luc and their weights measured every day. ( c ) Comparison of bioluminescence and viral copy number. Luciferase activities were quantified using ‘Living Image’ software, and quantitative RT-PCR were performed on RNA recovered from mouse lung homogenates. Each data point represents mean±s.e.m. (qRT-PCR n =3; luciferase n =7). Luciferase activity is expressed as p s −1 and viral copy number is expressed as arbitrary units (a.u.). Full size image To determine whether there was a direct correlation between the bioluminescence intensity and the viral titre in the lung, we collected the lungs from mice at days 3, 4, 5 and 7 p.i. and the viral load was measured by qRT-PCR and compared between the different viruses. We observed a good correlation (spearman r =0.941; P =0.017) between relative viral load in the lungs and bioluminescence intensity, validating the use of bioluminescence as a marker to assess the viral load in the lungs of mice infected with rHRSV-Luc ( Fig. 5c ). Together, these results show that bioluminescence imaging in rHRSV-Luc-infected mice reflects the status of pulmonary infection in real time. Real-time imaging of antiviral agent in vivo To test whether rHRSV-Luc can be used for in vivo assessment of antiviral drugs, AZD4316 was administered daily as a single oral 50-mg kg −1 dose and given 1 h prior to inoculation of virus at day 0, based on the efficacious dose and administration route established for this compound through in vivo study with wt RSV A2 (ref. 24 ). Mice were infected with 5 × 10 4 p.f.u. of rHRSV-Luc and in vivo bioluminescence intensity was determined daily ( Fig. 6 ). Bioluminescence was strongly reduced in the respiratory tract for mice treated with AZD4316 (159,200±13,636 photons (p) s −1 ), whereas mice that received no drug displayed strong bioluminescence (1.2 × 10 6 ±89,500 p s −1 ) ( Fig. 6a ). Very low signal (83,050 p s −1 ) was detected for mock-infected mouse. This result showed that rHRSV-Luc can be used as a tool for in vivo evaluation of drug efficiency against RSV using the mouse model. 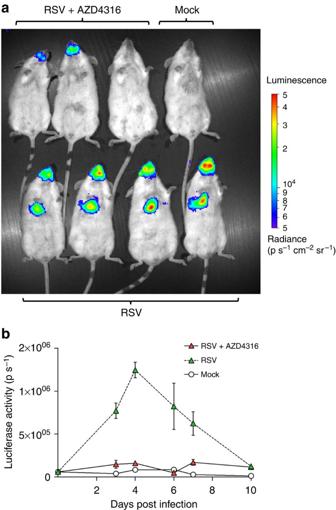Figure 6: Bioluminescence imaging of rHRSV-Luc allows evaluation of antiviral therapeutics in living mice. (a) Mice mock-infected (right mouse, upper panel) or infected with 5 × 104p.f.u. of rHRSV-Luc were untreated (lower panel) or treated with AZD4316 1 h prior to infection by oral gavage. Bioluminescence imaging of mice was analysed 3 days post infection as described inFig. 5. (b) Comparative time course of bioluminescence between AZD4316 and mock-treated mice. Each data point represents mean±s.e.m. (n=3). The statistical significance of differences were calculated using the Student’st-test. Figure 6: Bioluminescence imaging of rHRSV-Luc allows evaluation of antiviral therapeutics in living mice. ( a ) Mice mock-infected (right mouse, upper panel) or infected with 5 × 10 4 p.f.u. of rHRSV-Luc were untreated (lower panel) or treated with AZD4316 1 h prior to infection by oral gavage. Bioluminescence imaging of mice was analysed 3 days post infection as described in Fig. 5 . ( b ) Comparative time course of bioluminescence between AZD4316 and mock-treated mice. Each data point represents mean±s.e.m. ( n =3). The statistical significance of differences were calculated using the Student’s t -test. Full size image It is urgent to develop antiviral drugs and vaccines against RSV. Although several molecules have been shown to inhibit RSV replication in vitro (reviewed in ref. 28 ), currently none is available as a commercialized drug (reviewed in ref. 29 ). This is due at least in part to the cumbersome screening systems for RSV that moreover require biosafety level 2 confined facilities. We have developed a new reverse genetics system for RSV allowing easy manipulation of the genome by introducing enzyme restriction sites all along the cDNA in intergenic regions. This construct will allow the easy insertion of other reporter genes, or modifications of individual genes. Two recombinant RSV viruses, expressing either mCherry red fluorescent protein or firefly luciferase reporters, were derived from this construct. Replication rates of the three recombinant viruses, together with the WT virus (Long strain), were roughly similar, showing that the presence of foreign mCherry and Luc genes inserted between P and M transcription units had little effect on virus replication in vitro . Recombinant RSV viruses expressing GFP , beta-galactosidase , Katushka or R. luciferase foreign genes were previously constructed [8] . In most of these viruses, the reporter gene was placed at the 3′ end of the genome as the first gene expressed. However, van Remmerden et al . [30] noticed that a rHRSV with a EGFP gene placed upstream from NS1 was attenuated compared with a construct with the EGFP gene located between SH and G or WT virus. A similar result was obtained with beta-galactosidase [9] . Thus, it is likely that insertion of a supplementary gene at the first position is detrimental to the growth properties of RSV by decreasing or delaying the expression of NS genes, which was not observed with our constructs. Reporter gene expression was shown to mirror viral replication and can be used to monitor viral growth, eliminating the time-consuming fixation and staining steps as well as manual plaque counting. Using reporter gene expression inhibition, we found EC 50 values very similar to those determined with reference methods. These recombinant viruses may be reliable tools to study antiviral drugs for screening as well as advanced characterization. Each of these recombinants has its own advantages and disadvantages for automated high-throughput screenings. The rHRSV-Cherry virus requires a fluorescent plate reader but no consumable except plastic dishes and cell culture media. On the other hand, the rHRSV-Luc virus requires a luminometer and reaction substrates for the luciferase assay, and is thus more expensive, but also more sensitive and more accurate, with greater dynamic range and lower background. The rHRSV-Luc readout can also be performed on stored frozen plates (after cell lysis) for several days, allowing for batch analyses. It may also be coupled with a cell viability assay relaying on R. luciferase activity to assess both drug toxicity and efficacy in the same assay. Our recombinant RSVs, expressing either mCherry or firefly luciferase (Luc) have two advantages over other reporter constructs for both in vitro and in vivo studies. First, the background of red fluorescence is generally lower than for green fluorescence, particularly in organ tissues. Thus, rHRSV-Cherry could be useful for in vivo identification of target cells for RSV replication in the lung other than epithelial cells. Second, firefly Luc allows in vivo studies, as shown in this work, when using the BALB/c mouse model and a charge-coupled device camera, the consumables being relatively cheap. Compared with R. luciferase , the Luc activity is more stable, and the substrate can be administered by the nasal route. These two new recombinant viruses could constitute useful and complementary tools for future screening assays. Indeed, rHRSV-Cherry could be more convenient for the first steps of high-throughput screening assays, whereas rHRV-Luc should be more useful for precise determination of EC 50 and quantification of the exact level of RSV replication in the presence of drugs. More recently, a new technology allowing real-time tracking of cell invasion by RSV in cultured HEp-2 cells was described [31] . This technology is based on prior RSV surface labelling with biotin and revelation by gold nanoparticles combined to streptavidin using dark-field microscopy. Since gold-labelled RSV particles are still infectious, this approach is well adapted for studying the cell invasion process by RSV or its inhibition by drugs targeting the fusion process. However, in contrast to our recombinant viruses, this methodology cannot be applied to screening of drugs targeting the viral polymerase, large-scale screenings or in vivo studies. Mouse is the most popular species for experimental modelling of HRSV disease [7] . Here we have shown that the recombinant virus rHRSV-Luc can be used in living mice to monitor virus replication using a non-invasive imaging technique. Since luminescence was detected in all rHRSV-Luc-infected mice, and since the same living animal can be monitored at different time points, the number of animals needed to collect sufficient data can be reduced to 3 or 4 mice per experiment. This is to our knowledge the first report of in vivo imaging of RSV replication. RSV replication was detected in the snout and lungs of living mice, as previously described [32] . Since we used 10–1,000-fold-less infectious particles per mouse than usually used [7] , these results also show how sensitive the readout is for RSV replication using the Luc assay. Since clinical signs are very moderate in mice experimentally infected with HRSV, with low-to-moderate histopathology associated with moderate viral replication, our in vivo imaging technique adapted to RSV is a really powerful, practical and easy to use approach to follow RSV replication. Furthermore, it allows the release of laborious techniques such as qRT-PCR that requires animal killing. We have shown that mice infected with rHRSV-Luc can also be used as an animal model for testing antiviral drug efficacy. It is interesting that the RSV fusion inhibitor AZD4316 attenuated but did not completely block RSV replication in the nasopharynx of some of the mice tested under the experiment conditions. However, it was sufficient to stop the spread of RSV from nasopharynx to lung in all mice tested, reaching the goal of a successful RSV therapy, to prevent lower-respiratory tract infection. This result highlighted the potential to evaluate RSV treatment window, antiviral targets and points of intervention for efficacious therapy through monitoring the RSV replication kinetics and the time course of virus spread in the same animals using this non-invasive reporter virus system. In conclusion, these new tools constitute a powerful method not only to monitor viral replication in vivo in real time, but also for developing new therapeutic strategies. Our future challenge will be to improve this mouse model by increasing the capacity of these recombinant RSVs to replicate in mice and/or to induce clinical signs. This aim could be addressed by slotting in genes from other RSV strains or more recent isolates such as Line 19 (refs 33 , 34 ) or memphis 37 (ref. 35 ) more adapted for testing vaccines that aim to protect against currently circulating strains of RSV. Ethics statement This study was carried out in accordance with INRA guidelines in compliance with European animal welfare regulation. The protocols were approved by the Animal Care and Use Committee at ‘Centre de Recherche de Jouy-en-Josas’ (COMETHEA; protocol number 12–125) under relevant institutional authorization (‘Direction départementale de la Protection des Populations des Yvelines’, permit numbers: A78-167 and 78-27). All experimental procedures were performed in Biosafety level 2 facilities. Cells HEp-2 (ATCC number CCL-23) and BSRT7/5 (ref. 36 ) cells were maintained in Eagle’s minimum essential medium and Dulbecco’s modified Eagle’s medium, respectively, supplemented with 10% fetal calf serum, 2 mM L-glutamine, and penicillin–streptomycin solution. The cells were grown in an incubator at 37 °C in 5% CO 2 . Cytotoxicity assays were done with the CellTiter-Glo Luminescent cell viability assay (Promega) after 48 h of incubation with the compounds. Construction of HRSV cDNA clones To construct a full-length cDNA clone of HRSV subgroup A, strain Long (GenBank accession: AY911262), non-cutting enzymes (KpnI, BspEI, MluI, StuI, BstEII, SalI, BstBI), or unique cutting enzymes (XhoI, BamHI) in the HRSV cDNA were identified. A polylinker containing the designed restriction sites with a downstream HDV ribozyme sequence followed by a T7 transcription terminator, and an upstream T7 promoter was inserted into the low-copy vector pACNR1180 (ref. 22 ) (a kind gift of Dr Jon-Duri Tratschin, Institute of Virology and Immunoprophylaxis, Mittelhäusern, Switzerland) at the SmaI restriction site. Random-primed cDNA synthesis was done using SuperscriptII (Gibco-BRL) and 1 μg of total cytoplasmic RNA isolated from HEp-2 cells infected with the human RSV subgroup A, Long strain (ATCC VR-26). PCR was performed on cDNA using high-fidelity Pfu Ultra Polymerase (5U; Stratagene) and specific primers ( Table 1 ) to amplify 11 fragments covering the whole RSV genome (Genbank accession no. : AY911262.1) using standard procedures. The complete HRSV genome was sequenced using two independent PCR products for each fragment and was used as a reference. The BamHI and BstBI restriction sites present in the G cDNA sequence of our HRSV strain were destroyed by site-directed mutagenesis without modifying the amino-acid sequence. The KpnI, BspEI, MluI, StuI, BstEII and SalI restriction sites, absent from the HRSV cDNA, were placed in the NS2/N , N/P , P/M and G/M2 intergenic regions, respectively. Unique SacII and BstBI sites were introduced in the Leader and Trailer sequences, respectively, and a unique SalI site was placed into the variable region 2 of L [21] . The SacII site was destroyed thereafter by site-directed mutagenesis. The construction of a full-length HRSV cDNA clone resulted in a total of 16 nucleotide changes in the intergenic regions. The amplified fragments were cloned into separate pJET2.1 vectors (Fermentas) and the sequences were verified. The antigenomic cDNA spanning the entire HRSV genome was assembled into a single molecule by sequential ligation of RSV cDNA fragments into the pACNR1180-derived vector by standard subcloning techniques. The Leader end was constructed to abut the promoter for T7 RNA polymerase, and the Trailer end was constructed to be adjacent to the autocatalytic HDV ribozyme sequence. The resulting vector, pACNR–rHRSV, generates a positive sense, antigenomic RNA transcript with three additional G residues at its 5′ terminus, but leaving the exact 3′ native terminus. The positions and sequences of the alterations due to restriction site insertions are listed in Table 1 . Table 1 List of the primers used to construct the modified HRSV genome cDNA used in this work. Full size table The firefly luciferase (Luc) and mCherry genes were amplified by PCR using specific primers. The forward and reverse primers ( Table 1 ) were first flanked by the RSV gene start and gene end sequences from the HRSV P and N genes, respectively, and containing a MluI restriction site at the 5′ end to enable the insertion of the gene unit into the pACNR–rHRSV vector. All constructs were verified by sequencing. Transfection and recovery of recombinant viruses The reverse genetics vectors pACNR–rHRSV, pACNR–rHRSV-Cherry and pACNR–rHRSV-Luc (1.25 μg) were co-transfected together with the expression vectors p-N (1 μg), p-P (1 μg), p-L (0.5 μg) and p-M2-1 (0.25 μg), each under the control of the T7 promoter [21] in subconfluent BSR5T7/5 cells monolayers in 35-mm dishes, using 10 μl of FuGENE HD (Promega) reagent according to the manufacturer’s recommendations. Virus was collected at 72 h post transfection and titrated in plaque assay to assess virus rescue efficiency. The recombinant viruses were amplified on fresh HEp-2 cells at 37 °C at low multiplicity of infection (<0.01 p.f.u. per cell) for 3 days. RT-PCR was performed at passage 3 to verify the presence of the MluI restriction site in the P / M intergenic region of rHRSV. Virus stocks were frozen at passages 3 and 4. Virus titration by a plaque assay Viruses were titrated on HEp-2 cells at 37 °C using a plaque assay procedure adapted from Matrosovitch et al . [37] In brief, cells were infected with serial 10-fold dilutions of viral suspension in complete minimum essential medium (MEM). The overlay was prepared with microcrystalline cellulose Avicel RC581 (FMC Biopolymer) at a final concentration of 0.6% in complete MEM containing 1% fetal calf serum. After 6 days at 37 °C and 5% CO 2 , plaques were revealed by 0.5% crystal violet/20% ethanol solution staining of the cell layers, and the number of p.f.u. per well was counted by naked eye. rHRSV-Luc and rHRSV-Cherry titration assays HEp-2 cells were seeded at 5 × 10 4 cells per well in 96-well plates the day before, and infected with serially threefold-diluted viral suspensions beginning with 3,000–10,000 p.f.u. per well. For the mCherry assay, MEM without phenol red (Gibco) was used for cell culture and virus dilutions. For the luciferase assay, infected cells were incubated at 37 °C and 5% CO 2 for 24 h, then washed in 1 × phosphate-buffered saline (PBS) before lysis with 50 μl of lysis buffer (25 mM Tris pH 7.8, 8 mM MgCl 2 , 1% Triton X-100, 15% glycerol, 1 mM dithiothreitol) per well for 15 min at room temperature with gentle shaking. Plate and substrate were equilibrated at 37 °C before luciferase activity measurement, expressed in RLU using a Tecan infinite M200PRO plate reader and automatic injection for delivering 100 μl of 2 μM D -luciferin (Sigma) and ATP 10 mM in lysis buffer. For mCherry fluorescence measurement, infected cells were incubated at 37 °C and 5% CO 2 for 48 h. Fluorescence could be observed with a fluorescence microscope and was measured using a spectrofluorometer (Tecan infinite M200PRO) with excitation and emission wavelengths of 580 and 620 nm, respectively, (expressed in relative fluorescence units). Non-infected HEp-2 cells were used as standards for fluorescence and luminescence background levels. Plaque reduction assays For plaque reduction assays, the rHRSV-Cherry virus was grown on HEp-2 cells in the presence of serial threefold dilutions of the RSV polymerase inhibitor AZ-27 (refs 25 ) (27 μM to 4.1 nM) or the RSV fusion inhibitor BMS-433771 analogue AZD4316 (refs 23 , 24 ) (1,000–0.15 nM) and plaques were counted using the plaque assay protocol described above. The plaque numbers were plotted against the compound concentrations. EC 50 was graphically determined as the inhibitor concentration inducing 50% reduction of the plaque numbers. rHRSV-luciferase or rHRSV-mCherry inhibition assay HEp-2 cells were seeded at 5 × 10 4 cells per well in 96-well plates the day before and infected with 1,000 or 500 p.f.u. of RSV-luc or RSV-mCherry, respectively, in the presence of various drug concentrations. Compounds were solubilized at 10 mM in 100% v/v DMSO and further diluted in water to 1 mM, then serially diluted threefold in MEM without phenol red medium to final concentrations of 27 μM to 0.15 nM for AZ-27 and of 333 nM to 0.002 nM for AZD4316. DMSO dilutions in the same range as AZ-27 were also used as controls. Compound dilutions were pre-incubated with viral suspension for 5 min at 37 °C before addition on cell monolayers in 96-well plates. Plates were incubated at 37 °C for 24 h for rHRSV-Luc and 48 h for rHRSV-Cherry. Luciferase assay or mCherry fluorescence measurement was performed as described above. Luminescent readings and fluorescence readings are expressed as percentage of the mean control value (12 wells infected without drugs). EC 50 was calculated by fitting the data to sigmoidal curve equation (m1+(m2−m1) (1+( × m3 −1 )^m4) −1 using the Levenberg–Marquardt algorithm, as provided in the commercially available KaleidaGraph software package (Synergy Software). Mouse strains Female BALB/c mice were purchased from the Centre d'Elevage R. Janvier (Le Genest Saint-Isle, France) and were used around 8 weeks of age. Mice strains were bred in a pathogen-free animal facility. Mice were fed normal mouse chow and water ad libitum and were raised and housed under standard conditions with air filtration. For infection experiments, mice were housed in cages inside stainless steel isolation cabinets that were ventilated under negative pressure with high-efficiency particulate air-filtered air. Mouse infections Mice were anesthetized by a mixture of ketamine and xylazine (1 and 0.2 mg per mouse, respectively) and infected IN with 50 μl of PBS containing 6 × 10 4 p.f.u. of rHRSV-Luc. Body weight was monitored at days 3–10. For in vivo imaging, mice were anesthetized. Alternatively, mice were killed at different time points, and lungs were then collected. For each time point, experiments were done in triplicate. For antiviral drug administration to animals, AZD4316 was dissolved in sterile water at 5 mg ml −1 , and the solution was adjusted to pH 2.5 with HCl (0.1 N) as previously described [24] . All animals were treated with 0.2 ml of dissolved AZD4316, delivered by oral gavage. Oral treatments were administered 1 h prior to RSV inoculation and then once daily. RNA extraction and qRT-PCR analysis Viral loads were measured from lung homogenates by qRT-PCR. Briefly, lungs were crushed and total RNA was extracted from lung homogenates using the RNeasy mini kit (Qiagen) according to the manufacturer’s instructions. Four μg of individual RNA samples were reverse transcribed for 1 h at 42 °C, using 300 U of M-MLV Reverse Transcriptase (SuperScript II, Invitrogen) with 7 μM of random hexanucleotide primers (pd(N)6 (Pharmacia Biotech), 15 nmol of each deoxynucleotide triphosphate, 5 mM dithiothreitol and 60 U of ribonuclease inhibitor (RNaseOUT, Invitrogen) according to the manufacturer’s instructions. The primers (from Sigma–Aldrich, aliquoted and stored frozen as 100 μM solutions at −20 °C) used to target either the HRSV N gene or the murine HPRT gene have the following sequences: N forward primer, 5′- AGATCAACTTCTGTCATCCAGCAA -3′; N reverse primer, 5′- TTCTGCACATCATAATTAGGAGTATCAAT -3′; HPRT forward primer, 5′- CAGGCCAGACTTTGTTGGAT -3′; HPRT reverse primer, 5′- TTGCGCTCATCTTAGGCTTT -3′. Individual cDNA were mixed with SYBR GREEN PCR Master Mix (Life Technologies) with primers targeting the N gene or primers targeting the murine HPRT gene. Real-time PCR was run in 96-well microplates on Realplex Mastercycler (Eppendorf). For determination of the viral load or, individual cDNA (1 μl diluted in 10 μl RNAse-free water) were mixed with 15 μl SYBR GREEN PCR Master Mix (Applied Biosystems) containing 300 nM of both N primers, or 500 nM of both HPRT primers, in triplicate for each gene. Non-template controls were run in each assay. Fluorescence curves were analysed using the Realplex Mastercycler sequence detector (Eppendorf) to determine the cycle threshold (Ct) values for each gene. Individual data were normalized to HPRT by calculating the ΔCt value (Ct (N) median−Ct (HPRT) median). The relative quantity of N transcripts, normalized to HPRT, is expressed in a.u. In vivo luminescence measurements Mice were anaesthetized and luminescence was measured 5 min after IN or IP injection of 50 μl of PBS containing D -luciferin (Sigma) using 0.75 mg kg −1 for IN and 7.5 mg kg −1 for IP route. Photon emission of mock-infected and rHRSV-Luc-infected mice (6 × 10 4 p.f.u. per mouse) was measured using the IVIS 200 imaging system (Xenogen Corp.). Living Image software (version 4.0, Caliper Life Sciences) was used to measure the luciferase activities. Bioluminescence images were acquired for 1 min with f/stop=1 and binning=8. A digital false-colour photon emission image of the mouse was generated, and photons were counted within a constant region of interest corresponding to the surface of the chest encompassing the whole-airway area. Photon emission was measured as radiance in p s −1 cm −2 sr −1 . How to cite this article: Rameix-Welti, M.-A. et al . Visualizing the replication of respiratory syncytial virus in cells and in living mice. Nat. Commun. 5:5104 doi: 10.1038/ncomms6104 (2014). Accession codes: The nucleotide sequences of rHRSV, rHRSV-Luc and rHRSV-Cherry were deposited in the Genbank nucleotide database with accession codes KF713490 , KF713491 and KF713492 .